Ultra-sensitive liquid biopsy of circulating extracellular vesicles using ExoScreen Cancer cells secrete small membranous extracellular vesicles (EVs) into their microenvironment and circulation. Although their potential as cancer biomarkers has been promising, the identification and quantification of EVs in clinical samples remains challenging. Here we describe a sensitive and rapid analytical technique for profiling circulating EVs directly from blood samples of patients with colorectal cancer. EVs are captured by two types of antibodies and are detected by photosensitizer-beads, which enables us to detect cancer-derived EVs without a purification step. We also show that circulating EVs can be used for detection of colorectal cancer using the antigen CD147, which is embedded in cancer-linked EVs. This work describes a new liquid biopsy technique to sensitively detect disease-specific circulating EVs and provides perspectives in translational medicine from the standpoint of diagnosis and therapy. Cancer cells secrete various types of humoral factors into their microenvironment that are biomarkers for disease diagnosis and prognosis, including cytokines, chemokines and nucleic acids. Extracellular vesicles (EVs), including exosome and microvesicles from cancer cells, have also been found in the blood of cancer patients [1] , [2] , [3] , [4] , [5] , [6] , [7] and therefore provide a novel type of biomarker for various patient scenarios. EVs are small membranous vesicles that differ in their cellular origin, abundance and biogenesis [8] , and are naturally secreted by almost all cell types to transport bioactive molecules intercellularly. EVs are positive for tetraspanin family proteins, such as CD63, CD81 and CD9 (refs 9 , 10 , 11 ), and contain cell surface proteins as well as both mRNA and microRNA [12] . Conventional methods of analyzing EVs generally require large quantities of EVs to be concentrated and processed via time-consuming immunoblotting or enzyme-linked immunosorbent assay (ELISA) assays; these methods are impractical in most clinical settings. In this study, we establish a highly sensitive and rapid analytical technique for profiling surface proteins in EVs from patient blood that can be used to identify biomarkers of colorectal cancer, named ExoScreen. ExoScreen could monitor circulating EVs in serum without the need for purification step. In addition, we show that ExoScreen is superior for the detection of EVs to conventional methods, immunoblotting and ELISA. Furthermore, we find that ExoScreen enables to detect CD147 and CD9 double-positive EVs, which is abundantly secreted from colorectal cancer cells, in serum from colorectal cancer patients. Our results demonstrate that ExoScreen can be a tool for detection of EVs from as little as 5 μl of cancer patients’ serum to detect circulating cancer-derived EVs. Establishment of ExoScreen to detect EVs in serum To realize the usage of EVs in clinical situation, we develop methods that specifically detect circulating EVs in the serum based on an amplified luminescent proximity homogeneous assay using photosensitizer-beads [13] without a purification step of EVs ( Fig. 1 ). This system utilizes streptavidin-coated donor beads to capture an analyte-specific biotinylated antibody, and acceptor beads conjugated to a second antibody that recognizes an epitope of the analyte. The donor beads are excited with a laser at 680 nm, resulting in the release of singlet oxygen, which excites an amplified fluorescent signal in the acceptor beads. As a result, the acceptor beads emit light at 615 nm, but only if they are within 200 nm of the analyte captured by both antibodies. As shown in Fig. 2a , the size of EVs measured by the Nanosight particle tracking system was approximately 100 nm, which prevented the detection of larger vesicles, such as apoptotic bodies, shedding vesicles or protein complexes. In addition, we could not obtain signals from CD63 recombinant protein by ExoScreen, indicating that this assay does not detect antigen monomers ( Fig. 2b ). We call this assay ‘ExoScreen’ because the target of the assay is EVs and because it has a possibility to screen for biomarker of various diseases. 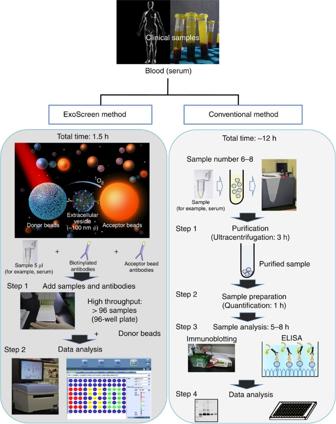Figure 1: Schematic overview depicting the method for detecting circulating EVs via conventional methods and ExoScreen. In the case of conventional methods, nearly 12 h are needed to detect the expression of certain protein in circulating EVs. In addition, excessive volumes of serum are required. Conversely, ExoScreen is completed within 2 h and requires only 5 μl of serum. In this system, streptavidin-coated donor beads capture an analyte-specific biotinylated antibody and are used in conjunction with acceptor beads conjugated to a second antibody. The streptavidin-coated donor beads are excited with a laser at 680 nm, resulting in the release of singlet oxygen, which excites an amplified fluorescent signal in the acceptor bead that emits at 615 nm when the beads are within 200 nm of the captured analyte. Figure 1: Schematic overview depicting the method for detecting circulating EVs via conventional methods and ExoScreen. In the case of conventional methods, nearly 12 h are needed to detect the expression of certain protein in circulating EVs. In addition, excessive volumes of serum are required. Conversely, ExoScreen is completed within 2 h and requires only 5 μl of serum. In this system, streptavidin-coated donor beads capture an analyte-specific biotinylated antibody and are used in conjunction with acceptor beads conjugated to a second antibody. The streptavidin-coated donor beads are excited with a laser at 680 nm, resulting in the release of singlet oxygen, which excites an amplified fluorescent signal in the acceptor bead that emits at 615 nm when the beads are within 200 nm of the captured analyte. 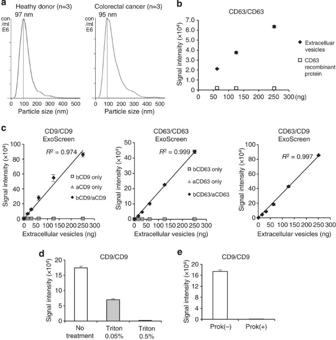Figure 2: Establishment of ExoScreen to detect the EVs. (a) Analysis of the size distribution in the serum of healthy donors (n=3) and colorectal cancer patients (n=3) by the NanoSight nanoparticle tracking system. (b) Detection of EVs or monomeric recombinant CD63 protein by ExoScreen using a CD63 antibody. EV protein concentration was measured via the Qubit system. The concentration of recombinant CD63 was adjusted with that of protein in EVs purified from HCT116 CM. Error bars are s.e.m. (n=3 for each condition). (c) Correlation between ExoScreen measurements for CD9 positive EVs, CD63 positive EVs or CD63/CD9 double-positive EVs and EV protein concentration in a dilution series. EV protein concentration was measured via the Qubit system. EVs were purified from HCT116 cell CM. The addition of biotinylated CD9 or CD63 antibodies without acceptor beads conjugated to antibodies is denoted ‘bCD9 only’ or ‘bCD63 only’, while ‘aCD9 only’ or ‘aCD63 only’ means addition of only acceptor beads conjugated to CD9 or CD63 antibodies without biotinylated antibodies. The addition of biotinylated antibodies and acceptor beads conjugated antibodies is denoted ‘bCD9/aCD9’ or ‘bCD63/aCD63’. Right panel shows the addition of biotinylated CD63 antibodies and acceptor beads conjugated CD9 antibodies. Error bars are s.e.m. (n=3 for each condition). (d) Evaluation of ExoScreen specificity against purified EVs from HCT116 cell treated with or without 0.05% and 0.5% Triton X-100. Two hundred fifty ng of EVs were detected by ExoScreen using CD9 antibodies. Error bars are s.e.m. (n=3 for each condition). (e) Evaluation of ExoScreen specificity against EVs from HCT116 cells treated with (Prok(+)) or without (Prok(−)) Proteinase K. Two hundred fifty ng of EVs were detected by ExoScreen using CD9 antibodies. Error bars are s.e.m. (n=3 for each condition). Data are representative of at least three independent experiments each. Full size image Figure 2: Establishment of ExoScreen to detect the EVs. ( a ) Analysis of the size distribution in the serum of healthy donors ( n =3) and colorectal cancer patients ( n =3) by the NanoSight nanoparticle tracking system. ( b ) Detection of EVs or monomeric recombinant CD63 protein by ExoScreen using a CD63 antibody. EV protein concentration was measured via the Qubit system. The concentration of recombinant CD63 was adjusted with that of protein in EVs purified from HCT116 CM. Error bars are s.e.m. ( n =3 for each condition). ( c ) Correlation between ExoScreen measurements for CD9 positive EVs, CD63 positive EVs or CD63/CD9 double-positive EVs and EV protein concentration in a dilution series. EV protein concentration was measured via the Qubit system. EVs were purified from HCT116 cell CM. The addition of biotinylated CD9 or CD63 antibodies without acceptor beads conjugated to antibodies is denoted ‘bCD9 only’ or ‘bCD63 only’, while ‘aCD9 only’ or ‘aCD63 only’ means addition of only acceptor beads conjugated to CD9 or CD63 antibodies without biotinylated antibodies. The addition of biotinylated antibodies and acceptor beads conjugated antibodies is denoted ‘bCD9/aCD9’ or ‘bCD63/aCD63’. Right panel shows the addition of biotinylated CD63 antibodies and acceptor beads conjugated CD9 antibodies. Error bars are s.e.m. ( n =3 for each condition). ( d ) Evaluation of ExoScreen specificity against purified EVs from HCT116 cell treated with or without 0.05% and 0.5% Triton X-100. Two hundred fifty ng of EVs were detected by ExoScreen using CD9 antibodies. Error bars are s.e.m. ( n =3 for each condition). ( e ) Evaluation of ExoScreen specificity against EVs from HCT116 cells treated with (Prok(+)) or without (Prok(−)) Proteinase K. Two hundred fifty ng of EVs were detected by ExoScreen using CD9 antibodies. Error bars are s.e.m. ( n =3 for each condition). Data are representative of at least three independent experiments each. Full size image To confirm the reliability for detecting EVs by ExoScreen, we selected CD9 and CD63, which are abundant on the surface of EVs and are expressed in numerous cells, to detect EVs. Conditioned medium (CM) of prostate cancer, prostate epithelial, breast cancer and colorectal cancer cell lines were processed to obtain purified EVs. ExoScreen was able to quantify the amount of EVs present in cell culture supernatants with CD9 and CD63 positive EVs detectable in a dose-dependent manner ( Fig. 2c and Supplementary Fig. 1 ). The negative controls, represented by only the biotinylated antibody or acceptor bead-conjugated antibody, resulted in a minimal fluorescent signal ( Fig. 2c ). In addition, the signal was decreased after detergent treatment ( Fig. 2d and Supplementary Fig. 2 ) or Proteinase K treatment ( Fig. 2e and Supplementary Fig. 3 ), indicating that ExoScreen detected complexes of membranous vesicle and transmembrane proteins. Immunoblotting of the same purified EVs preparations confirmed the data obtained by ExoScreen. In fact, CD9 and CD63 proteins were detectable via immunoblotting ( Fig. 3a and Supplementary Fig. 4 ). As shown in Fig. 3a , approximately 32 ng of EV proteins were needed to properly detect CD63 by immunoblotting, while ExoScreen could detect 15.6 ng of purified EVs ( Fig. 2c ). Furthermore, EVs from only 1 μl of culture medium are enough to detect by ExoScreen ( Fig. 3b and Supplementary Fig. 5 ). In addition, ExoScreen has a wide working range compared with ELISA ( Figs 2c and 3c ). Moreover, because ExoScreen is a mix-and-read assay, these conventional methods require many steps and substantial time compared with ExoScreen ( Fig. 1 ). Thus, the ExoScreen assay increases throughput while substantially decreasing hands-on. Taken together, these results indicate that ExoScreen is superior for the detection of EVs to conventional immunoblotting and ELISA ( Table 1 ). The results of EVs detection in culture supernatant without purification ( Fig. 3b , Supplementary Figs 5 and 6 ) prompted us to investigate whether ExoScreen could detect and characterize EVs in human serum. To develop ExoScreen as a diagnostic tool for clinical use, we optimized the method to detect EVs in serum without purification because the protocol exhibited non-linearity of ExoScreen signals against serum samples ( Fig. 4a ). This non-linearity is most likely a result of the aggregation of condensed proteins in serum. Indeed, we added dextran-500 to suppress serum protein aggregation, and this treatment eliminated the disruption of signals by protein aggregation ( Fig. 4a ). As shown in Fig. 4a , ExoScreen revealed that serum EVs were captured and expressed both CD9 and CD63 without purification. Further, these signals were detectable in a dose-dependent manner ( Fig. 4a ). In addition, we assessed whether the concentration of beads, which we employed in this study, was appropriate for the detection of circulating EVs in serum by checking the various concentrations of beads via ExoScreen, and found that the concentration of beads we employed in this study was adequate ( Fig. 4b ). Taken together, these results indicated that ExoScreen could monitor circulating EVs in serum without the need for a purification process. 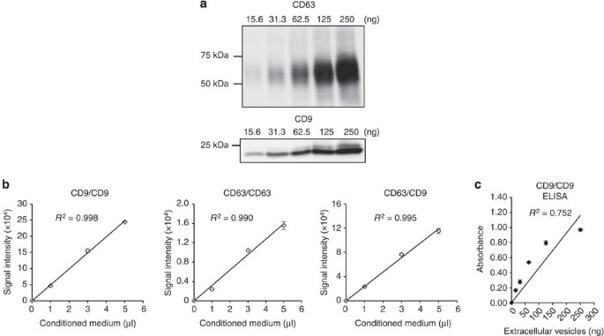Figure 3: Comparison of ExoScreen and conventional methods. (a) Immunoblotting analysis of CD63 (upper panels) or CD9 (lower panels) against the EVs isolated from HCT116 cells. EV protein concentration were measured via the Qubit system. EVs were purified from HCT116 cell CM. (b) Correlation between ExoScreen measurements for CD9 positive, CD63 positive or CD63/CD9 double-positive EVs and HCT116 cell CM in a dilution series. CM was prepared for 5 μl and diluted as indicated. Error bars are s.e.m. (n=3 for each condition). (c) Correlation between ELISA measurements for CD9 positive EVs and EV protein concentration in a dilution series. EV protein concentration were measured via the Qubit system. EVs were purified from HCT116 cell CM. Error bars are s.e.m. (n=3 for each condition). Data are representative of at least three independent experiments each. Figure 3: Comparison of ExoScreen and conventional methods. ( a ) Immunoblotting analysis of CD63 (upper panels) or CD9 (lower panels) against the EVs isolated from HCT116 cells. EV protein concentration were measured via the Qubit system. EVs were purified from HCT116 cell CM. ( b ) Correlation between ExoScreen measurements for CD9 positive, CD63 positive or CD63/CD9 double-positive EVs and HCT116 cell CM in a dilution series. CM was prepared for 5 μl and diluted as indicated. Error bars are s.e.m. ( n =3 for each condition). ( c ) Correlation between ELISA measurements for CD9 positive EVs and EV protein concentration in a dilution series. EV protein concentration were measured via the Qubit system. EVs were purified from HCT116 cell CM. Error bars are s.e.m. ( n =3 for each condition). Data are representative of at least three independent experiments each. Full size image Table 1 Comparison of ExoScreen and ELISA. 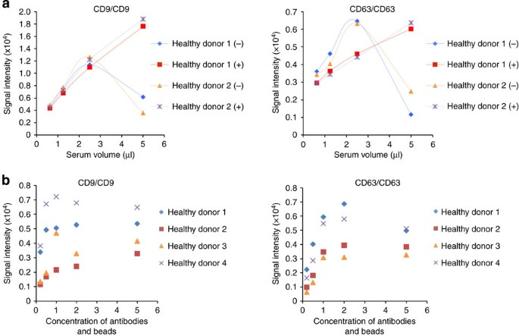Figure 4: Detection of circulating EVs in healthy donor sera. (a) Correlation between ExoScreen measurements for CD9 or CD63 and serum volume in a dilution series with (+) or without (−) Dextran-500. The final concentration of Dextran-500 was 1 mg ml−1. (b) Concentration of ‘1’ means the original concentration of donor and acceptor beads which we used in this study (see Methods section). In addition to original concentration, increased (twofold and fivefold) and decreased (0.5-fold and 0.25-fold) amount of donor and acceptor beads were evaluated by ExoScreen using serum from four healthy donors. Data are representative of at least three independent experiments each. Full size table Figure 4: Detection of circulating EVs in healthy donor sera. ( a ) Correlation between ExoScreen measurements for CD9 or CD63 and serum volume in a dilution series with (+) or without (−) Dextran-500. The final concentration of Dextran-500 was 1 mg ml −1 . ( b ) Concentration of ‘1’ means the original concentration of donor and acceptor beads which we used in this study (see Methods section). In addition to original concentration, increased (twofold and fivefold) and decreased (0.5-fold and 0.25-fold) amount of donor and acceptor beads were evaluated by ExoScreen using serum from four healthy donors. Data are representative of at least three independent experiments each. Full size image Enrichment of CD147 on EVs from colorectal cancer cell lines Because EVs are known to represent an important and specific route of intercellular communication [14] , we reasoned that tumour-derived EVs may differ from circulating EVs in normal physiological conditions. Previous reports showed that the protein components of EVs from cancer cells were different from normal cells [15] , [16] . Indeed, it has been recently reported that for patients with stage III melanoma, the amount of specific protein in EVs was significantly increased in individuals who eventually developed metastatic disease, indicating that EVs might have great potential for cancer diagnosis [6] . To identify cancer-derived EVs in cancer patients, EVs derived from the colorectal cancer cell line HCT116 cells and a normal colon fibroblast cell line CCD-18Co cells were subjected to proteomic analysis ( Supplementary Table 1 ). When EVs isolated from CCD-18Co cells were compared with HCT116 cells, the amount of CD147, which is the immunoglobulin superfamily member, was found to be significantly high in the EVs of HCT116 cells, whereas the expression could not be observed in CCD-18Co cells. Notably, CD147 is plasma membrane protein and this is suitable for applying to the ExoScreen. We observed that CD147 is expressed on all of the colorectal cancer cell lines, but their expression levels are not uniform ( Fig. 5a,b and Supplementary Figs 7 and 8 ). In addition, CD147 in EVs from CCD-18Co cells was hardly detectable. Several reports have shown that CD147 is expressed in the majority of human tumour types including colorectal cancer [17] , [18] , although CD147 is expressed in a variety of embryonic and adult tissues, such as spermatocytes, neuronal cells, erythrocyte and so on [19] . In addition, CD147 functions in lactate transporter, which is an important feature of cancer cell, because of the excessive anaerobic glycolysis phenomenon in cancer cells referred to as the Warburg effect [20] . Indeed, associations between high expression of CD147 and poor prognosis have previously been shown in colorectal cancer [21] , thus representing a potential marker for ex vivo analysis of tumour-derived EVs. 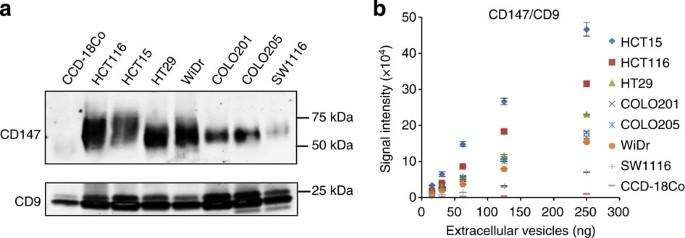Figure 5: Analysis of the amount of CD147 in EVs derived from various colon cancer cell lines and a normal colon fibroblast cell line. (a) Immunoblotting analysis of CD147 or CD9 against purified EVs isolated from CCD-18Co cells, HCT116 cells, HCT15 cells, HT29 cells, WiDr cells, COLO201 cells, COLO205 cells and SW1116 cells. EV proteins (250 ng) was used for the detection of CD147 and CD9. (b) Correlation between ExoScreen detection of CD147/CD9 double-positive EVs and EV protein concentration in a dilution series. EVs protein concentration was measured via the Qubit system. EVs were purified from CCD-18Co, HCT116, HCT15, HT29, WiDr, COLO201, COLO205 or SW1116 CM. Error bars are s.e.m. (n=3 for each condition). Data are representative of at least three independent experiments each. Figure 5: Analysis of the amount of CD147 in EVs derived from various colon cancer cell lines and a normal colon fibroblast cell line. ( a ) Immunoblotting analysis of CD147 or CD9 against purified EVs isolated from CCD-18Co cells, HCT116 cells, HCT15 cells, HT29 cells, WiDr cells, COLO201 cells, COLO205 cells and SW1116 cells. EV proteins (250 ng) was used for the detection of CD147 and CD9. ( b ) Correlation between ExoScreen detection of CD147/CD9 double-positive EVs and EV protein concentration in a dilution series. EVs protein concentration was measured via the Qubit system. EVs were purified from CCD-18Co, HCT116, HCT15, HT29, WiDr, COLO201, COLO205 or SW1116 CM. Error bars are s.e.m. ( n =3 for each condition). Data are representative of at least three independent experiments each. Full size image CD147 and CD9 double-positive EVs in clinical samples Next, we used ExoScreen to detect cancer-derived EVs in human clinical samples ( Fig. 6a ). As shown in Fig. 6a , we found that CD147 and CD9 double-positive EVs were significantly higher in serum from cancer patients ( n =194) than in serum from healthy donors ( n =191). Most importantly, most of CD147 in cancer patient sera reduced after surgery ( Fig. 6b ), suggesting that the reduced signal of CD147 obtained from ExoScreen is originated from cancer-derived EVs, even the variety of cells expressed CD147. To confirm whether by ExoScreen really reflects the protein profile of EVs in circulation, EVs were purified from the sera of tumour patients ( n =35) and healthy donors ( n =10) and analysed for expression of CD147 via immunoblotting ( Supplementary Fig. 9 ). We also performed ExoScreen against the same serum samples obtained by ultracentrifugation ( Fig. 6c , right panel). As depicted in Supplementary Fig. 9 , the expression of CD147 in EVs isolated from the sera of cancer patients correlated clearly with the results obtained from the ExoScreen assay ( Fig. 6c ), indicating that the accuracy of ExoScreen was confirmed and that it can be used to monitor EVs in circulation without any purification. Taken together, these results demonstrate that ExoScreen can be a tool for detection of EVs from as little as 5 μl of cancer patients’ serum to detect circulating cancer-derived EVs. 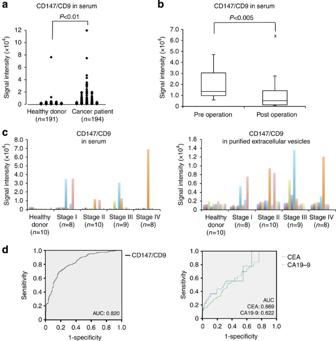Figure 6: Analysis of circulating CD147 and CD9 double-positive EVs in healthy donors or colorectal cancer patient sera. (a) Serum levels of CD147/CD9 double-positive EVs in colorectal cancer patients without any purification. The panel shows a scatter plot for healthy donors (n=191) and colorectal cancer patients (n=194). TheP-value was calculated by using Wilcoxon rank-sum test. (b) Changes in serum levels of CD147/CD9 double-positive EVs in colorectal cancer patients (stage I or II:n=15) before (preoperation) and after (postoperation after 7–34 days) surgical removal of the tumor. Box lengths represent the interquartile range (first to third quartiles). The line in the center of the boxes represents the median value. Data represented by the asterisks are extreme values (greater than three times the interquartile range over the third quartile). TheP-value was calculated by using Wilcoxon signed-rank test. (c) The results of ExoScreen detection of circulating EVs (left panel) and purified circulating EVs (right panel) in sera from healthy donors (n=10) and colorectal cancer patients (n=35) using CD147 and CD9 antibodies. The panels show the signal intensities from each samples measured for CD147/CD9 double-positive EVs using ExoScreen. (d) Receiver operating characteristic curves between healthy donors and colorectal cancer patients assesing by CD147/CD9 double-positive EVs (left panel), CEA and CA19-9 (right panel). left panel, CD147/CD9 double-positive EVs (healthy donors versus colorectal cancer patients; AUC: 0.820); right panel, CEA (AUC: 0.669); CA19-9 (AUC: 0.622) Data are representative of at least three independent experiments each. AUC, area under the curve. Figure 6: Analysis of circulating CD147 and CD9 double-positive EVs in healthy donors or colorectal cancer patient sera. ( a ) Serum levels of CD147/CD9 double-positive EVs in colorectal cancer patients without any purification. The panel shows a scatter plot for healthy donors ( n =191) and colorectal cancer patients ( n =194). The P -value was calculated by using Wilcoxon rank-sum test. ( b ) Changes in serum levels of CD147/CD9 double-positive EVs in colorectal cancer patients (stage I or II: n =15) before (preoperation) and after (postoperation after 7–34 days) surgical removal of the tumor. Box lengths represent the interquartile range (first to third quartiles). The line in the center of the boxes represents the median value. Data represented by the asterisks are extreme values (greater than three times the interquartile range over the third quartile). The P -value was calculated by using Wilcoxon signed-rank test. ( c ) The results of ExoScreen detection of circulating EVs (left panel) and purified circulating EVs (right panel) in sera from healthy donors ( n =10) and colorectal cancer patients ( n =35) using CD147 and CD9 antibodies. The panels show the signal intensities from each samples measured for CD147/CD9 double-positive EVs using ExoScreen. ( d ) Receiver operating characteristic curves between healthy donors and colorectal cancer patients assesing by CD147/CD9 double-positive EVs (left panel), CEA and CA19-9 (right panel). left panel, CD147/CD9 double-positive EVs (healthy donors versus colorectal cancer patients; AUC: 0.820); right panel, CEA (AUC: 0.669); CA19-9 (AUC: 0.622) Data are representative of at least three independent experiments each. AUC, area under the curve. Full size image In summary, we propose a rapid, highly sensitive and widely usable detection method based on the amplified luminescent proximity homogeneous assay using photosensitizer-beads for cancer cell-derived EVs. Notably, different antibodies can be conjugated to capture different analytes, such as CD147, thus various types of cancer can be targetd. There are various colorectal cancer screening tests. For example, the fecal occult blood test has been recommended widely as a screening test for colorectal cancer; however, the fecal occult blood displays low sensitivity and specificity for detecting colorectal cancer [22] . Moreover, carcinoembrionic antigen (CEA) and carbohydrate antigen 19-9 (CA19-9) are the most commonly used tumour-associated antigens in the management of patients with colorectal cancer, although those biomarkers are not sensitive enough for early colorectal cancer [23] , [24] . In fact, the high levels of CD147 detected in patient sera showed the normal value range of CEA and CA19-9 in stage I patients ( Supplementary Tables 2 and 3 ). In addition, the receiver operating characteristic curve indicates a diagnostic advantage of CD147/CD9 double-positive EVs in comparison with CEA and CA19-9 ( Fig. 6d ). From these aspects and the result shown in Fig. 6b , ExoScreen detecting CD147/CD9 double-positive EVs might be used for monitoring the status of cancer after the surgery and during chemotherapy, resulting in increase in QOL of the patients and providing doctor for the proper assessment of patient status. Further studies are needed to know whether our ExoScreen reduces colorectal cancer mortality as a screening test. It should be noted that CD147/CD9 double-positive EVs were also detected in samples with early stage colorectal cancer that invade into submucosal layer (T1 stage according to UICC classification) ( Supplementary Table 2 ) by the ExoScreen assay. These results also indicate that ExoScreen can be used to detect biomarkers for diseases that are currently difficult to diagnose and monitor not only cancer, but autoimmune disease and degenerative disease of the brain. Thus, our data suggest that ExoScreen, in addition to being a novel liquid biopsy platform for the detection of circulating EVs, may aid variety of disease diagnosis and help to identify companion biomarkers that are important for new drug development. Cell cultures Human colorectal cancer cell lines (HCT116 cells, HCT15 cells, HT29 cells, COLO201 cells, COLO205 cells, WiDr cells and SW1116 cells) and normal colon fibroblast cell line CCD-18Co cells were purchased from American Type Culture Collection. HCT116 and HT29 cells were cultured in McCoy’s 5A medium supplemented with 10% heat-inactivated fetal bovine serum (FBS) and an antibiotic–antimycotic solution (Invitrogen) at 37 °C in 5% CO 2 . WiDr cells CCD-18Co cells were cultured in minimal essential medium (MEM) containing 2 mM L -gulutamine, an antibiotic–antimycotic solution, nonessential amino acids and 10% FBS at 37 °C in 5% CO 2 . HCT15 cells, COLO201 cells and COLO205 cells were cultured in RPMI 1640 medium supplemented with 10% heat-inactivated FBS and an antibiotic–antimycotic solution at 37 °C in 5% CO 2 . SW1116 cells were cultured in Leibovitz’ L15 medium supplemented with 10% heat-inactivated FBS and an antibiotic–antimycotic solution at 37 °C in without CO 2 . The following additional cell lines were used: PNT2 cells, an immortalized normal adult prostatic epithelial cell line (DS Pharma Biomedical Co., Ltd. Osaka, Japan); PC3 cells, a human prostate cancer cell line initiated from a bone metastasis of a grade IV prostatic adenocarcinoma (American Type Culture Collection); MDA-MB-231-luc-D3H2LN cells (MDA-MB-231LN), a highly metastatic human breast cancer cell line (Xenogen); and MCF7 cells, a human breast cancer cell line which expresses oestrogen receptor (American Type Culture Collection). The above cells were cultured in RPMI 1640 medium supplemented with 10% FBS and an antibiotic–antimycotic solution at 37 °C in 5% CO 2 . Patient serum samples Collection and usage of human serum from corolectal cancer patients ( n =194) and healthy donor ( n =94) were approved by Osaka university Institutional Review Board (No.11343). Serum was aliquoted and kept at −80 °C until used, and freeze-thawing was avoided as much as possible after that. Some part of the serum samples ( n =97) from healthy donor shown in Fig. 6a were purchased from BizCom Japan (Tokyo, Japan). Serum samples containing red blood cells were excluded from the analysis. Informed consent was obtained from all patients. Preparation of conditioned media and EVs The cells were washed with phosphate-buffered saline (PBS), and the culture medium was replaced with advanced Dulbecco’s Modified Eagle Medium for HCT116 cells, WiDr cells, SW1116 cells, HT29 cells and CCD-18Co cells, or advanced RPMI medium for the other cell lines, containing an antibiotic–antimycotic and 2 mM L -glutamine (but not containing FBS). After incubation for 48 h, the CM was collected and centrifuged at 2,000 g for 10 min at 4 °C. To thoroughly remove cellular debris, the supernatant was filtered through a 0.22 μm filter (Millipore). The CM was then used for EV isolation. To prepare EVs, CM or the sera from colorectal patients and healthy donors were ultracentrifuged at 110,000 g for 70 min at 4 °C. The pellets were washed with 11 ml of PBS, ultracentrifuged at 110,000 g for 70 min at 4 °C and resuspended in PBS. The putative EVs fraction was measured for its protein content using a Quant-iT Protein Assay with Qubit2.0 Fluorometer (Invitrogen). Reagents The following antibodies were used for immunoblotting: mouse monoclonal anti-human CD63 antibody (clone H5C6, dilution 1:200) from BD Biosciences, mouse monoclonal anti-human CD9 antibody (clone ALB 6, dilution 1:200) from SantaCruz Biotechnology, mouse monoclonal anti-human CD147 antibody (clone MEM-M6/1, dilution 1:1,000) from Novus Biologicals and mouse monoclonal anti-Actin (clone C4, dilution 1:1,000) from Millipore. The secondary antibody (horseradish peroxidase-labeled sheep anti-mouse) were purchased from GE HealthCare. The following antibodies used for ExoScreen and ELISA were developed in Shionogi & Co., LTD.: mouse monoclonal anti-human CD63 antibody (clone 8A12) and mouse monoclonal anti-human CD9 antibody (clone 12A12). Mouse monoclonal anti-human CD147 antibody (clone MEM-M6/1) was purchased from Novus Biologicals. Antibodies were used to modify either acceptor bead or biotin following the manufacturer’s protocol. AlphaLISA reagents (Perkin Elmer, Inc., Waltham, MA 02451, USA) consisted of AlphaScreen Streptavidin-coated donor beads (6760002), AlphaLISA Unconjugated-acceptor beads (6062011) and AlphaLISA Universal buffer (AL001F). AlphaLISA assays were performed in 96-well half-area white plates (6005560) and read in an EnSpire Alpha 2300 Multilabel Plate reader (Perkin Elmer, Inc.). ExoScreen assay A 96-well half-area white plate was filled with 5 μl of sample, 5 nM biotinylated antibodies and 50 μg ml −1 AlphaLISA acceptor beads conjugated antibodies in the universal buffer. The volume of each reagent was 10 μl. The plate was then incubated for 1–3 h at room temperature. Without a washing step, 25 μl of 80 μg ml −1 AlphaScreen streptavidin-coated donor beads were added. The reaction mixture was incubated in the dark for another 30 min at room temperature and the plate was then read on the EnSpire Alpha 2300 Multilabel Plate reader using an excitation wavelength of 680 nm and emission detection set at 615 nm. Background signals obtained from PBS were subtracted from the measured signals. ELISA Ninety-six well-plates (Nunc) were coated with 2.5 μg ml −1 anti-human CD9 or -CD63 antibodies in a volume of 50 μl per well of carbonate buffer (pH 9.6) and incubated for 4 h at room temperature. After 2 washes with 0.01% Tween-20 in PBS, 100 μl per well of Blocking One solution (Nacalai Tesque) was added at room temperature for 1 h. Following 3 washes in PBS, EVs purified from cell culture supernatants were added in a final volume of 50 μl and incubated for 1 h at room temperature. After 3 washes with PBS, 50 μl of biotinylated anti-human CD9 or -CD63 antibodies diluted to 1 μg ml −1 were added and incubated for 1 h at room temperature. After 3 washes with PBS, the plate was incubated with 100 μl of HRP-conjugated streptavidin (Cell Signalling Technology) diluted 1:2,000 in Blocking One solution for 1 h at room temperature. After the final 3 washes with PBS, the reaction was developed with Peroxidase (TMB One Component HRP Microwell Substrate, SurModics). The reaction was arrested with 450 nm Stop Reagent for TMB Microwell Substrates (SurModics) and optical densities were recorded at 450 nm. Immunoblotting Equal amounts of EVs or whole-cell lysates were loaded onto 4–15% Mini-PROTEAN TGX gels (Bio-Rad, Munich, Germany). Following electrophoresis (100 V, 30 mA), the proteins were transferred to a polyvinylidene difluoride membrane. The membranes were blocked with Blocking One solution and then incubated with primary antibodies. After washing, the membranes were incubated with horseradish peroxidase-conjugated sheep anti-mouse IgG and then subjected to enhanced chemiluminescence using ImmunoStar LD (Wako). CD63, CD9 and CD147 were detected under non-reducing conditions. Original scans of the cropped images in the main figures ( Figs 3a and 5a ) are presented in Supplementary Fig. 10 . Measurement of size distribution by NTA Nanoparticle tracking analysis (NTA) was carried out using the Nanosight system (NanoSight) on sera diluted 1000-fold with PBS for analysis. The system focuses a laser beam through a suspension of the particles of interest. These are visualized by light scattering using a conventional optical microscope aligned perpendicularly to the beam axis, which collects light scattered from every particle in the field of view. A 60 s video recorded all events for further analysis by NTA software. The Brownian motion of each particle was tracked between frames to calculate its size using the Stokes–Einstein equation. How to cite this article: Yoshioka, Y. et al . Ultra-sensitive liquid biopsy of circulating extracellular vesicles using ExoScreen. Nat. Commun. 5:3591 doi: 10.1038/ncomms4591 (2014).